Acute emergence and reversion of influenza A virus quasispecies within CD8+T cell antigenic peptides Influenza A virus-specific CD8 + cytotoxic T lymphocytes (CTLs) provide a degree of cross-strain protection that is potentially subverted by mutation. Here we describe the sequential emergence of such variants within CTL epitopes for a persistently infected, immunocompromised infant. Further analysis in immunodeficient and wild-type mice supports the view that CTL escape variants arise frequently in influenza, accumulate with time and revert in the absence of immune pressure under MHCI-mismatched conditions. Viral fitness, the abundance of endogenous CD8 + T cell responses and T cell receptor repertoire diversity influence the nature of these de novo mutants. Structural characterization of dominant escape variants shows how the peptide–MHCI interaction is modified to affect variant-MHCI stability. The mechanism of influenza virus escape thus looks comparable to that recognized for chronic RNA viruses like HIV and HCV, suggesting that immunocompromised patients with prolonged viral infection could have an important part in the emergence of influenza quasispecies. Quasispecies capable of rapid adaptation to selection pressures are characteristic of infections with persistent RNA viruses such as the human immunodeficiency virus (HIV) and hepatitis C virus (HCV). Such variation occurs both within the antibody-binding [1] , [2] sites on viral proteins and in the peptide+class I MHC glycoprotein (pepMHCI) epitopes [3] , [4] recognized by CD8 + cytotoxic T lymphocytes (CTLs). However, while the regular emergence of ‘seasonal’ influenza viruses reflects the selection of antibody escape mutants of the surface hemagglutinin (HA) and neuraminidase (NA) molecules [5] , the viral components of the pepMHCI CTL antigenic regions are generally thought to be more conserved. The difference may be that influenza is normally an acute and readily resolved infection, whereas HCV and HIV have evolved to cause sustained viremia in the presence of an ongoing antibody response. Any influenza pepMHCI mutants may be rapidly neutralized by the HA-specific immunoglobulin (Ig) response. When a novel pandemic or seasonal influenza A virus emerges and evades pre-existing antibody immunity, established CD8 + T cell memory to conserved viral regions can potentially ameliorate the consequences of human exposure. Influenza-specific CTLs mediate the acute clearance of infection from the lung and, when recalled from memory, provide some protection against novel strains sharing internal peptides but expressing different HA and/or NA molecules [6] , [7] . It is thus possible that at least one component of a future, cross-protective influenza vaccine might be focused on developing substantial CTL memory populations. Prior to designing such a vaccine, however, we need to develop a clearer picture of influenza peptide conservation. There is some evidence for virus evasion of CD8 + CTL immunity for both naturally occurring variants (from databases of consensus sequences) and from experiments with chronically infected transgenic mice [8] , [9] , [10] , though both the part played by CTL-mediated immune pressure and the prevalence of viable mutants in nature merit further analysis. Here we analyse the evolution of influenza CTL variants for longitudinally isolated viruses from an unusual human case and in RNA samples from influenza virus-infected mouse lungs. This characterization of variants from an immunocompromised patient with a prolonged influenza virus infection provides the first documented series showing the ‘natural’, sequential evolution of influenza quasispecies within human CTL antigenic regions, similar to those observed for HIV [11] and SHIV [12] . A well-established lung infection model in immune-deficient (Ig −/− or Ig −/− CTL −/− ) and wild type (wt) C57Bl/J (B6, H2 b ) mice was then used to dissect the parameters influencing the emergence of such novel influenza virus variants, with the key peptide changes then being compared at the structural level. Apart from providing clear evidence that influenza variants readily emerge and accumulate with time in this acute virus infection, the present analysis illuminates the nature of immune escape at a molecular level. Furthermore, the fact that such mutants revert to the wild-type (wt) sequence in MHCI-mismatched animals where there is no immune pressure reflects that these changes in key antigenic peptides make the viruses less fit, as further supported by our experimental data. Variations in CTL epitopes thus occur as readily for acute influenza as for chronic HIV and HCV, though their emergence for influenza in immunocompetent individuals is likely limited by a normal, concurrent Ig response. Evolution of quasispecies in persistent human influenza Sequential influenza A virus (H3N2) isolates were obtained from an infant [13] who received multiagent chemotherapy for acute B-cell lymphoblastic leukaemia at 9 weeks post-partum. First infected at 1 year, the H3N2 virus persisted for 12 months (August 1997–August 1998), presenting one of the longest reported influenza cases to date [13] . Perhaps due to CTL-mediated clearance, the infection terminated spontaneously during a temporary cessation of chemotherapy [13] . Previous characterization of the surface HA and NA glycoproteins showed rates of antigenic drift comparable to those found at the population level for circulating H3N2 influenza viruses. Taking advantage of the unique resource offered by these sequential viral isolates from a single individual, we searched for changes in the immunogenic nucleoprotein (NP) and matrix 1 protein (M1) candidate pepMHCI CTL epitopes. Based on the patient’s HLA types (HLA-A*A0201/HLA-A*3101, HLA-B*8/HLA-B*27), we compared the viral peptides presented by the relevant MHCIs (Immune Epitope Database http://www.iedb.org ) [14] , [15] over the period of influenza virus infection. 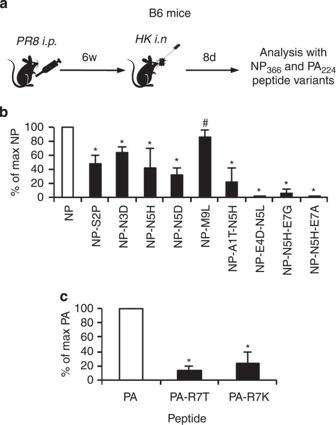Figure 1: Reduced recognition ofde novomutants by wt-specific CTL responses. (a) Splenic lymphocytes recovered following secondary infection (wt-PR8→wt-HK) were assessed for recognition of the selected NP366and PA224peptide variants. Diminished recognition of the (b) NP366and (c) PA224variants (described inTable 2) by wt-specific CD8+CTLs. Cells were stimulated with wt-NP366/PA224(white bars) or a panel of mutant NP366/PA224peptides (black bars) and IFN-γ production was measured by a standard ICS assay. Data are represented as mean±s.d. forn=5. Each experiment was repeated at least twice.#P≤0.05, *P≤0.01 relative to wt DbNP366+and DbPA224+CD8+response (by a Student’st-test, two-tailed distribution). Our analysis showed sequence variation within 6/30 of the immunogenic pepMHCI candidates, three within M1 and three within NP ( Table 1 ; Supplementary Table S1 ). The gradual emergence of de novo variants is illustrated by two amino acid (aa) changes in the M1 129–137 (ASCMGL I Y N R→ASCMGL L Y S R) and M1 125–134 (GL I Y N RMGA→GL L Y S RMGA) peptides and one aa change in M1 178–187 (RMVLAS T TAK→RMVLAS I TAK). Importantly, our analysis of all the documented epitope regions within NP and M1 revealed collectively nine mutations, with 78% of those ( n =7) occurring within the epitopes restricted by HLAs related to the patient. One mutation occurred within a suggested antigenic region of unknown HLA (M1 95–112 ) and one mutation was found in an epitope of unrelated HLA restriction (NP 17–25 restricted by HLA-B*4401, HLA-B*4002 and HLA-B*4501). Thus, our data suggest preferential emergence of the viral variants within epitopes restricted to this patient’s HLAs. The dominance of the mutants over the wt-virus increased after each round of antiviral therapy, suggesting that, if a variant is not eliminated by drug treatment, the outgrowth of mutant over wt may be intensified when the pathogen re-emerges. What surprised us is that the evolution of CTL variants within the one individual during a persistent influenza virus infection can be comparable to that found for immunosuppressive retroviruses in HIV-infected people [11] or SHIV-infected macaques [12] . Table 1 Emergence of influenza quasispecies in CTL antigenic regions during a persistent influenza infection in an immunocompromised patient. Full size table Emergence of influenza variants in immunocompromised mice Our findings on the sequential emergence of influenza mutants in the longitudinal samples obtained from an immunocompromised child provided physiological importance for the subsequent dissection of viral escape mutants in a mouse model of influenza infection. To investigate how mutants emerge under conditions of antibody compromise, T cell-competent Ig −/− μMT mice [16] were first primed intraperitoneally (i.p.) with the PR8 (H1N1) influenza virus and, together with T/B cell-deficient RAG −/− mice [17] that had been engrafted with polyclonal D b NP 366 + CD8 + memory T cells, were challenged intranasally (i.n.) with the HK (H3N2; shares PR8 internal proteins) virus. These two experimental designs ( Supplementary Fig. S1 ) probed the interplay between the emergence of viral variants in acute influenza infection and delayed virus clearance [18] in the context of immune pressure exerted by epitope-specific CD8 + CTLs. Lungs were sampled on d15, the latest time-point at which antigen is detectable in wt-B6 (H2 b ) mice [19] . Viral RNA was extracted and the NP 366 and PA 224 regions were amplified, cloned and sequenced. 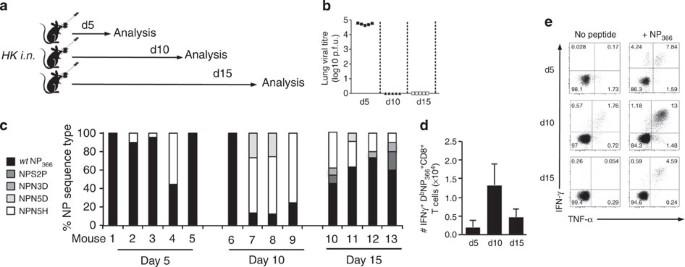Figure 2: Accumulation of NP366variants over time in unmanipulated wt mice. (a) Naive wt B6 mice were infected i.n. with wt HK virus at d0 and lungs were harvested on d5, d10 and d15. RNA was extracted and the NP366peptide region was amplified, cloned and sequenced. (b) Infectious virus titres were assessed using a standard plaque assay. (c) Prevalence of variant NP366peptide sequences are shown as the mutation frequency (%) for total recovered sequences. Data are derived from three different timepoints, and each mouse has repeated sequences from at least three RT–PCR of the NP vRNA. The NP366peptide region of the input HK viral stock was sequenced with no mutations being isolated. (d,e) The DbNP366+CD8+T cell responses in BAL (n=5; mean±s.d.) on d5, d10 and d15 were assessed by ICS. The experiment was repeated twice. Sequencing the input wt-PR8 and wt-HK viruses confirmed the clonality of the wt-NP 366 and wt-PA 224 sequences ( Table 2 , Supplementary Table S2 ). However, viral RNA recovered from the lungs of all three RAG −/− mice on d15 contained multiple NP 366–374 variants ( Table 2 ). The most striking results were in mouse (m) 3, where 100% of the NP 366 sequences were mutated, predominantly at position (P) 5 (NP-N5H), the H2D b peptide anchor [20] , [21] . The most prominent mutation (NP-N5H) was then associated with various secondary changes (at P1, P4 and P7) and mutations outside the immunogenic peptide region ( Supplementary Table S3 ) that may further disrupt peptide presentation or overcome the fitness costs associated with NP-N5H. Furthermore, the D b NP 366 + CD8 + response in m3 (9.2 × 10 3 cells) was three to six times larger than that for m1 (5.1 × 10 2 cells) and m2 (3.2 × 10 3 cells), suggesting that the dominance of the NP-N5H variant in m3 could result from a more pronounced D b NP 366 + CD8 + response exerting greater immune pressure on the virus. Of course, as the RAG −/− mice were given polyclonal, tetramer-sorted D b NP 366 + CD8 + CTLs, only the NP 366 peptide was targeted for escape. Table 2 De novo mutations are selected for NP 366 during infection of immune-compromised D b+ mice (as described Supplementary Fig. S1 ). Full size table The PR8-primed μMTs established CD8 + CTL responses to both D b NP 366 and D b PA 224 . Again, the NP-N5H variant (range: 8–33%) was found in all three mice (m4–6) with detectable viral RNA ( Table 2 ), and additional mutations were found at P2, P3 and P7. Previously, P3 was identified as a partially solvent exposed residue within D b NP 366 and the NP-N3A mutation was associated with a ~25% reduction in recognition by wt-D b NP 366 + CD8 + CTLs [18] . Furthermore, mutations at NP-S2P and NP-N3D decrease the pepMHCI affinity by 500 and 18 times, respectively [22] . In contrast, analysis of the PA 224 sequences from μMT mice showed much less evidence of adaptation ( Table 2 ), with only one variant (at P7) being selected. As the P7 of PA 224 is the most solvent-exposed residue for this MHC-I epitope [21] , the selection of PA-R7K would reduce wt-D b PA 224 + CD8 + CTL recognition. The difference in mutational frequency for these two epitopes could either reflect that D b NP 366 (but not D b PA 224 ) [23] is expressed on productively infected lung epithelium at a higher level or be a consequence of the greater D b PA 224 TCRβ repertoire diversity [22] , [23] , [24] . Recognition of variants by wt-CD8 + CTLs Does the preferential emergence of selected de novo variants with mutations at MHCI anchor residues reflect evasion of the wt epitope-specific CD8 + CTL response? Spleen cells from secondary-stimulated (HK→PR8) wt-B6 (H2 b ) mice were stimulated in vitro with the wt and mutant NP 366 and PA 224 peptides (identified in Table 2 ) and analysed for IFNγ production ( Fig. 1a ). Recognition of all the NP 366 variants by the wt-D b NP 366 + CD8 + CTLs was reduced ( Fig. 1b ) and while the response to NP-M9L was close to that for the wt-peptide (86±10% of the wt, P =0.036), this mutation may still confer some selective advantage. Surprisingly, the most prevalent NP-N5H variant did not completely compromise binding to H-2D b (at high peptide concentration of 1 μM, although had markedly reduced binding at lower peptide concentrations; Supplementary Fig. S2 ) and could be seen by some wt-D b NP 366 + CTLs (43±27% of wt), though co-mutations within NP 366 (at P1, P4 or P7 plus NP-N5H) were minimally recognized by the wt-responders ( Fig. 1b ). Furthermore, de novo variants ( Table 2 ) in PA 224 at P7 (PA-R7T and PA-R7K) were poorly recognized ( Fig. 1c ). Additional functional avidity analysis by peptide titration and probing with a hybridoma expressing a D b NP 366 -specific ‘public’ TCR ( Supplementary Fig. S2 ) further indicated that these de novo mutations in antigenic peptides are likely to confer selective advantage in the face of an ongoing, wt-CD8 + CTL response, with reduced avidity and recognition by a clonal TCR. Figure 1: Reduced recognition of de novo mutants by wt-specific CTL responses. ( a ) Splenic lymphocytes recovered following secondary infection (wt-PR8→wt-HK) were assessed for recognition of the selected NP 366 and PA 224 peptide variants. Diminished recognition of the ( b ) NP 366 and ( c ) PA 224 variants (described in Table 2 ) by wt-specific CD8 + CTLs. Cells were stimulated with wt-NP 366 /PA 224 (white bars) or a panel of mutant NP 366 /PA 224 peptides (black bars) and IFN-γ production was measured by a standard ICS assay. Data are represented as mean±s.d. for n =5. Each experiment was repeated at least twice. # P ≤0.05, * P ≤0.01 relative to wt D b NP 366 + and D b PA 224 + CD8 + response (by a Student’s t -test, two-tailed distribution). Full size image Evolution of de novo NP 366 variants in intact mice The findings in the immunocompromised, persistently infected infant and the frequent detection of influenza virus variants in the Ig −/− (but CTL-competent) μMT and CTL-reconstituted RAG −/− mice suggest that, in the absence of neutralizing antibody, escape occurs readily for some of the key peptides recognized by immune T cells. What happens when the antibody response is intact? Lungs from naive, wt-B6 mice ( Fig. 2a ) were analysed at d5, d10 and d15 following primary i.n. infection with the HK virus. Virus titres were high on d5, as expected [24] , and no infectious virus was recovered from d10–d15 ( Fig. 2b ). However, viral RNA [19] was detected on d15, with evidence of cumulative NP 366 sequence diversity ( Fig. 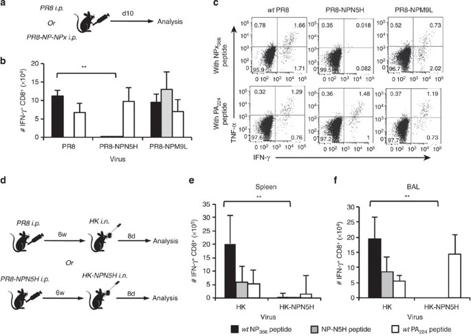Figure 3: Lack of CD8+T cell responses to the dominant NP-N5H escape variants. (a) Mice were primed i.p. with the wt PR8 or the PR8-NP-N5H or PR8-NP-M9L viruses (generated by reverse genetics) and spleens were isolated 10 days later. Cells were stimulated on a short-term with the wt NP366(black), NP-M9L or NP-N5H (grey) or PA224(white) peptide. Cytokine production was measured in a standard ICS assay. (b) The numbers of peptide-specific CD8+T cells were calculated from the % IFN-γ+CD8+T cells and the total cell counts. (c) Representative CD8+T cell IFN-γ and TNF-α ICS FACS plots; (d) Secondary CTL responses in mice (mean±s.d.,n=5) primed i.p. with either the wt PR8 or PR8-N5H virus were measured in (e) spleen and (f) BAL populations on d8 following i.n. challenge with the homologous HK variant. *P≤0.01 and **P≤0.001 relative to the wt DbNP366+CD8+T cell response (by a Student’st-test, two-tailed distribution). Data are represented as mean±s.d. forn=5. Each experiment was repeated at least twice. 2c , Table 3 ). The NP-N5H mutation was found as early as d5 (3/5 mice, range: 5–55%), increased till d10 (3/4 mice, 65±8%) and was present in all 4 mice on d15 (24±12%) with there being 2–3 mutant sequences per mouse. The NP-N5D variant identified here was previously isolated at low frequency (6% of sequences) from D b NP 366 TCR transgenic mice [25] . In m11, the NP-N5H and NP-N5D mutations were isolated in 27 and 9% of sequences, with both occurring as a single nucleotide change at P1 of the codon from N: A AC to H: C AC or D: G AC. Thus, NP-N5H must have a selective advantage over NP-N5D. Overall, our data from different experimental approaches provide clear evidence for the emergence of viral mutants within NP 366 on d15 after infection, with 7/9 mutants being found at the anchor residues (especially P5N). Furthermore, at d15 after infection, the mutation rates in the wt B6 mice (27–54%) and immunocompromised μMT mice (8–44%) were comparable ( P =0.27). Thus, immune escape within the NP 366 viral peptide occurs at similar frequency in both an intact and B cell-compromised immune system. Figure 2: Accumulation of NP 366 variants over time in unmanipulated wt mice. ( a ) Naive wt B6 mice were infected i.n. with wt HK virus at d0 and lungs were harvested on d5, d10 and d15. RNA was extracted and the NP 366 peptide region was amplified, cloned and sequenced. ( b ) Infectious virus titres were assessed using a standard plaque assay. ( c ) Prevalence of variant NP 366 peptide sequences are shown as the mutation frequency (%) for total recovered sequences. Data are derived from three different timepoints, and each mouse has repeated sequences from at least three RT–PCR of the NP vRNA. The NP 366 peptide region of the input HK viral stock was sequenced with no mutations being isolated. ( d , e ) The D b NP 366 + CD8 + T cell responses in BAL ( n =5; mean±s.d.) on d5, d10 and d15 were assessed by ICS. The experiment was repeated twice. Full size image Table 3 NP 366 mutations emerge over the course of infection of B6 mice (see Fig. 2c ), whereas the NP 147 ( K d ) peptide remains stable. Full size table Day 5 is the first time-point when influenza-specific CD8 + T cells can be recovered from the site of infection [26] , coincident with the emergence of mutant RNAs ( Fig. 2b,c,e ). Earlier analysis [27] showed that the D b NP 366 + CD8 + CTL response is fully recruited from the naive pool by d5, with peak numbers in the bronchoalveolar lavage (BAL) on d10, followed by contraction by d14–d15 (refs 24 , 28 ), a profile that is replicated here ( Fig. 2d,e ). The role of D b NP 366 + CTLs in providing the selective pressure that leads to the emergence of the influenza virus variants ( Fig. 2c , Table 3 ) is clear, as no mutations from the same mice were detected for the immunogenic NP 147–154 peptide presented by H2K d ( Table 3 ), an MHCI allele not expressed in B6 mice but associated with a strong response in the BALB/c strain. Any selective pressure manifesting as differential RNA diversity for peptides that bind H2D b versus H2K d must be reflective of live virus variant selection. Further sequencing of the viral PA 224–236 from B6 mice showed a low level of mutation (2.6±5.8%; Supplementary Table S4 ) compared with the 40.25±11.5% variability for the viral NP 366–374 ( P <0.001). This confirms that the D b NP 366 + CD8 + CTLs are more efficient at selecting mutant peptides. CD8 + CTL responses to engineered NP 366 variant viruses To determine how the selected mutations in NP 366 have an impact on influenza virus viability and the host CD8 + CTL response, key RNA variants were engineered into the PR8 backbone using a reverse genetic strategy [29] . High-titre PR8-NP-N5H and PR8-NP-M9L viruses were used to prime B6 mice via the non-replicative i.p. route ( Fig. 3a ) to exclude any effect due to differential virus growth. Using the D b PA 224 -specific response as an internal control ( Fig. 3b–f ), the PR8-NP-N5H virus did not elicit detectable CTLs for either the wt -D b NP 366 or the (notional) D b NP-N5H epitope ( Fig. 3b,c ). In addition, though secondary challenge (HK i.n.→PR8 i.p.) of wt-mice generated CTLs that responded in vitro following stimulation with the NP-N5H peptide ( Fig. 1b ), performing the same experiment with the PR8-NP-N5H and HK-NP-N5H engineered viruses gave no evidence for the generation of D b NP-N5H-specific CTLs ( Fig. 3d,e ). Thus, though D b NP-N5H can be recognized in vitro at a high peptide concentration, the NP-N5H anchor peptide must significantly reduce presentation in vivo , suggesting an explanation for the emergence of this variant. Conversely, the D b NP-M9L + CTL expansion following PR8-NP-M9L infection was equivalent to that found for the wt-D b NP 366 + CD8 + set in PR8-immune mice ( Fig. 3b ), indicating that these readily detected mutant RNAs are consequences of virus replication rather than immune selection, as NP-M9L is a rare variant ( Table 2 ) that could be eliminated by the wt-D b NP 366 + CTLs. Figure 3: Lack of CD8 + T cell responses to the dominant NP-N5H escape variants. ( a ) Mice were primed i.p. with the wt PR8 or the PR8-NP-N5H or PR8-NP-M9L viruses (generated by reverse genetics) and spleens were isolated 10 days later. Cells were stimulated on a short-term with the wt NP 366 (black), NP-M9L or NP-N5H (grey) or PA 224 (white) peptide. Cytokine production was measured in a standard ICS assay. ( b ) The numbers of peptide-specific CD8 + T cells were calculated from the % IFN-γ + CD8 + T cells and the total cell counts. ( c ) Representative CD8 + T cell IFN-γ and TNF-α ICS FACS plots; ( d ) Secondary CTL responses in mice (mean±s.d., n =5) primed i.p. with either the wt PR8 or PR8-N5H virus were measured in ( e ) spleen and ( f ) BAL populations on d8 following i.n. challenge with the homologous HK variant. * P ≤0.01 and ** P ≤0.001 relative to the wt D b NP 366 + CD8 + T cell response (by a Student’s t -test, two-tailed distribution). Data are represented as mean±s.d. for n =5. Each experiment was repeated at least twice. Full size image Reduced stability of the novel pepMHC complexes The impact of the peptide mutants on the integrity of the pepMHCI complexes was assessed by thermostability-based assays ( Supplementary Table S5 ). The wt-NP 366 and NP-N3D peptides are broadly equivalent in their capacity to stabilize the H2D b molecule, whereas stability is greatly reduced for the dominant anchor mutants, NP-N5D and NP-N5H. This is consistent with the inability of NP-N5H to induce either primary or secondary CTL responses ( Fig. 3 ). In order to illuminate the structural mechanisms underlying this decreased thermostability and viral escape, the structures for H2D b bound to NP-N5D, NP-N5H and NP-N3D were solved at a resolution of 1.9 Å, 2.2 Å and 2.8 Å, respectively ( Supplementary Table S5 ). Overall, the structures of the D b -binding cleft plus the three variant peptides were similar to that found for the wt-NP 366 (r.m.s.d.<0.6 Å) ( Fig. 4 ). As the NP 366 and NP-N3D are equivalent in their capacity to stabilize the D b molecule, it was no surprise that the D b NP-N3D MHC cleft was similar to that found for the D b NP 366 complex ( Fig. 4a ). In contrast, the P5-Histine side-chain within NP-N5H caused a restructuring of the cleft floor residues ( Fig. 4b,c ). While the P5-Asn of the wt-NP 366 hydrogen bonds to Gln97, the larger side chain of the P5-His pushes Gln97 away in order to fit inside the cleft as an anchor residue. Additionally, the conformations of Gln70 and His155 were both affected by the P5 mutation, with the consequence being increased flexibility. Thus, the P5 Asp→His mutation induced structural rearrangements needed to accommodate the large side chain of the P5-His, consistent with lower stability for the D b NP-N5H complex. Surprisingly, the P5-Asn mutation to a negatively charged P5-Asp resulted in two differing conformations of the peptide ( Fig. 4d,f ). One conformation was similar to the wt-NP 366 (r.m.s.d. of 0.42 Å) ( Fig. 4d ), in which the N5D mutation caused the peptide to sit deeper in the cleft and caused structural rearrangements of Gln97 and His155 ( Fig. 4e ). The alternate conformation exhibited a flip in the orientation of P5-P6, whereby the P5-Asp was solvent-exposed and the important TCR contact P6-Met [21] , [30] was partially buried ( Fig. 4f,g ) (r.m.s.d. of 1.11 Å). The dual conformations observed for the NP-N5D peptide reflected the high flexibility of this mutant, consistent with the reduced stability of the D b NP-N5D complex. 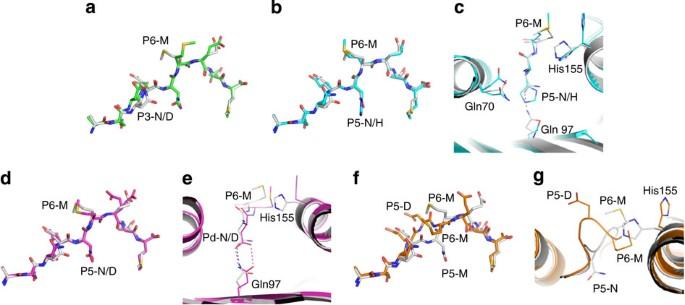Figure 4: The NP-N5H and NP-N5D variants show perturbed pepMHCI binding. (a,b) The structural superposition of the Db-bound wt NP366(white stick) peptide with NP-N3D (green) and NP-N5H (cyan stick) respectively. (c) Superposition of DbNP366(white) with the DbNP-N5H (cyan), with the Dbmolecule represented in cartoon, the peptide in stick and the black dashed lines represent the interactions made by NP366. (d,e) Superposition of DbNP366(white) and the first molecule of the DbNP-N5D (pink) structure, which is the most similar to the NP366peptide. (d) represents the peptide as stick and (e) shows the effect of the P5 residue mutation on the H2Dbmolecule (cartoon) and peptide (stick). The dashed line represents the interaction made by the Dbmolecule with either the NP366(black) or the NP-N5D peptide (pink). (f,g) Superposition of the DbNP366(white) and the second molecule of the Db-NP-N5D (orange) structure, being the alternate conformation of the NP-N5D peptide. (f) represents the peptide as stick and (g) shows the effect of the P5 residue mutation on the Dbmolecule (cartoon) and peptide (stick). Figure 4: The NP-N5H and NP-N5D variants show perturbed pepMHCI binding. ( a , b ) The structural superposition of the D b -bound wt NP 366 (white stick) peptide with NP-N3D (green) and NP-N5H (cyan stick) respectively. ( c ) Superposition of D b NP 366 (white) with the D b NP-N5H (cyan), with the D b molecule represented in cartoon, the peptide in stick and the black dashed lines represent the interactions made by NP 366 . ( d , e ) Superposition of D b NP 366 (white) and the first molecule of the D b NP-N5D (pink) structure, which is the most similar to the NP 366 peptide. ( d ) represents the peptide as stick and ( e ) shows the effect of the P5 residue mutation on the H2D b molecule (cartoon) and peptide (stick). The dashed line represents the interaction made by the D b molecule with either the NP 366 (black) or the NP-N5D peptide (pink). ( f , g ) Superposition of the D b NP 366 (white) and the second molecule of the D b -NP-N5D (orange) structure, being the alternate conformation of the NP-N5D peptide. ( f ) represents the peptide as stick and ( g ) shows the effect of the P5 residue mutation on the D b molecule (cartoon) and peptide (stick). Full size image Thus, both N5D and N5H escape variants induced structural rearrangements, which resulted in increased flexibility of those variant peptides within MHCI, consistent with lower stability of the overall D b NP-N5D/H complexes. This provides one possible explanation of why N5D/H-MHCI complexes do not induce TCR responses while still binding to the MHCI, albeit with increased flexibility and thus reduced stability. This is consistent with the inability of NP-N5H to induce either primary or secondary CTL responses. Reversion of NP-N5H in the absence of selective pressure Experimental evidence ( Figs 2 , 3 , 4 ) indicates that the preferential emergence of the dominant NP-N5H mutation reflects both diminished recognition by D b NP 366 + CTLs and the lack of an endogenous D b NP-N5H-specific response due to reduced MHCI binding. Reversion of unfit mutations to wt-sequence in naive MHCI-mismatched hosts is common [31] , [32] , reflecting the absence of the immune pressure that caused the initial emergence of the variant epitope. However, if replicative fitness is not severely impaired and the selective advantage is sufficient then the mutation can become fixed in nature [10] , [33] , [34] . To determine whether the PR8-NP-N5H mutant would revert to wt-NP 366 when MHCI is mismatched, BALB/c (H-2 d ) mice were infected with the engineered PR8-NP-N5H virus. The NP 366 region of the input PR8 and PR8-NP-N5H virus stocks were sequenced prior to infection and no mutations were detected ( Supplementary Table S2 ). Separate groups of BALB/c mice were then challenged i.n. with the PR8-NP-N5H or wt-PR8 virus and the NP 366 sequences were analysed on d15 ( Fig. 5a ). In all 5 BALB/c mice infected with PR8-NP-N5H virus, the wt-NP 366 sequence dominated (range: 57–100%) ( Fig. 5b , Supplementary Table S2 ). Thus in the absence of immune pressure from D b NP 366 + CD8 + CTLs, the NP-N5H sequence reverted to wt. This reversion of NP-N5H was not 100%, as the NP-N5H variant was still isolated in m1 and m2 (17 and 43%). Thus, in a natural transmission setting, the NP-N5H mutation might still be propagated to other hosts [31] . Unexpectedly, the NP-N3D sequence was generated de novo in m3, despite the input PR8-NP-N5H virus being 100% NP-N5H in sequence. This low-frequency isolation of NP-N3D in 1 of 10 mice infected with PR8-NP-N5H virus suggests the random isolation of the N3D mutant. Importantly, the NP-N3D mutation in MHC-mismatched Balb/C mice was found at a much lower rate than in B6 mice, in which the NP-N3D variant was isolated in three out of five mice on d15 after wt influenza virus infection ( Fig. 2c , Table 2 ). 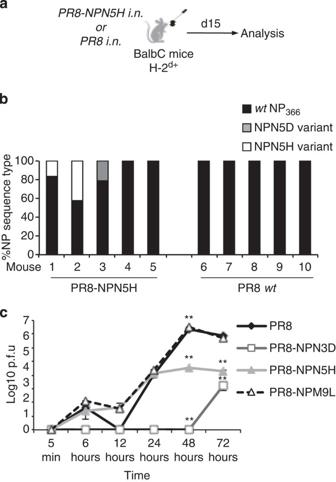Figure 5: The NP-N5H variant reverts to the wt-NP366in the absence of immune selection pressure. (a) MHCI-mismatched BALB/c (H-2d) mice were infected i.n. with engineered PR8-NP-N5H or wt PR8 viruses and RNA was extracted on d15. The NP366peptide region was amplified by PCR, cloned and sequenced. (b) show the NP366peptide sequences isolated after PR8-NP-N5H and PR8 infection (see alsoSupplementary Table S2). The NP366peptide regions of the input PR8-NP-N5H and PR8 virus stocks were sequenced and found to be homogeneous. Data represent the mutation frequency (%) of total sequences; m, mouse. (c) To assess replicative fitness, MDCK monolayers were infected with the wt PR8 (rescued by reverse genetics, black) or mutant PR8-NP viruses (dark grey/light grey/white) at an MOI of 0.01. Culture supernatants were harvested at various times from 5 min to 72 h. Data are represented as the mean±s.d. (n=3) in duplicate. **P≤0.001 and##P≤0.005 relative to wt PR8 virus (by a Student’st-test, two-tailed distribution). The results were reproduced in independent experiments using FOCI and HA assays as readouts. Figure 5: The NP-N5H variant reverts to the wt-NP 366 in the absence of immune selection pressure. ( a ) MHCI-mismatched BALB/c (H-2 d ) mice were infected i.n. with engineered PR8-NP-N5H or wt PR8 viruses and RNA was extracted on d15. The NP 366 peptide region was amplified by PCR, cloned and sequenced. ( b ) show the NP 366 peptide sequences isolated after PR8-NP-N5H and PR8 infection (see also Supplementary Table S2 ). The NP 366 peptide regions of the input PR8-NP-N5H and PR8 virus stocks were sequenced and found to be homogeneous. Data represent the mutation frequency (%) of total sequences; m, mouse. ( c ) To assess replicative fitness, MDCK monolayers were infected with the wt PR8 (rescued by reverse genetics, black) or mutant PR8-NP viruses (dark grey/light grey/white) at an MOI of 0.01. Culture supernatants were harvested at various times from 5 min to 72 h. Data are represented as the mean±s.d. ( n =3) in duplicate. ** P ≤0.001 and ## P ≤0.005 relative to wt PR8 virus (by a Student’s t -test, two-tailed distribution). The results were reproduced in independent experiments using FOCI and HA assays as readouts. Full size image Importantly, no mutations were found within viral NP 366-374 in BALB/c mice infected with the wt-PR8 virus, providing further evidence that the emergence of NP-N5H is driven by immune pressure from D b NP 366 + CD8 + CTLs. To determine viral fitness, MDCK monolayers were infected at an MOI of 0.01 over a time course with the main variants (NP-N5H, NP-N3D and NP-M9L) from H2 b mice ( Fig. 5c ). The PR8-NP-N3D virus was only detectable at 72 h after infection, whereas PR8-NP-N5H replicated but to a significantly lower titre than the wt-PR8 at 48–72 h. Thus, though the NP-N3D and NP-N5H mutations emerge due to immune pressure, they are less fit than the wt-virus. Selection of viral mutants is likely to be different when antibodies specific for surface glycoproteins (like influenza HA) rather than CTLs (specific for influenza MHCI-NP) are supplying the evolutionary pressure. When the NP mutation occurs in a productively infected cell, any newly released infectious virus variants may be readily neutralized by wt-HA-specific antibody. As a consequence, the likelihood that a CTL-selected mutant will emerge is greatly increased when humoral immunity is defective, and the opposite is true for HA variants. In the immunosuppressed (by chemotherapy) infant analysed here, it is significant that both the HA and CTL variants were detected in recovered, infectious virus. In nature, highly immunosuppressed humans (like those with untreated AIDS) with a profile of prolonged influenza infection (and thus viral shedding) may thus represent a major risk factor for the emergence of novel, seasonal influenza viruses. Currently, there are no data on the evolution of influenza viruses in AIDS patients, although clinical trials are underway in South Africa on influenza infections in individuals infected with HIV-1. Virus-specific CD8 + CTL-mediated immune escape during chronic HCV and HIV infections and with tumor-specific immunity [4] , [35] is associated with continued immune pressure. With HIV and SIV, CTL-selected variants may not appear immediately. Escape from the immunodominant Mane-A*10-KP9 + CTL response occurs between 2–11 weeks after infection [36] , whereas HIV variants selected by HLA-B44-gp160 30–38 -specific CTLs emerge within 6 weeks [4] . Influenza viruses, however, cause acute, localized infections that are normally cleared within 14 days [24] , [37] . Mouse experiments indicate that influenza infections of the respiratory tract can be terminated by CD8 + CTLs functioning in the absence of an Ig response or by high quality CD4 + ‘T-helped’ antibodies where CD8 + CTL-mediated immunity is compromised [38] . Even so, influenza virus control is optimal when all components of the immune response are operating. In the immunocompromised infant, CTL variants were found among six candidate peptides (relevant to this patient’s HLAs). As expected, no mutations were detected in the highly conserved [9] immunodominant HLA-A*0201-M1 58 epitope. Furthermore, the same was true for the variable HLA-B*27-NP 383 epitope, as the infecting influenza virus already contained NP 383 in its ‘escape anchor version’ (SGYWAIRTR) [39] , with co-mutations (E375G and M239V) present in the flanking residues that compensate for any loss of viral fitness [33] . The B*27-NP 383 anchor mutation is reminiscent of, or in some senses comparable to, the prevalent mouse D b -NP-N5H escape variant from our experimental study, whereby an anchor mutation has become fixed in seasonal isolates leading to the loss of an immunogenic peptide from the available pool of T cell antigens. Importantly, prior priming with the PR8-NP-N5H virus, and the subsequent recall with the HK-NP-N5H virus, was unable to overcome this virus escape mechanism, unlike the stimulation for escape at TCR contact residues [40] . As a consequence, the generation of anchor escape variants should be avoided by vaccination procedures that use viral peptides or live viruses. In the well-characterised B6 influenza model, antigenic variation in the PA 224 peptide was less common than for NP 366 , supporting previous findings of a correlation between viral escape and TCR repertoire diversity [41] . It is possible that the wt-D b PA 224 + CD8 + CTLs recognize emerging peptide variants via a diverse TCRβ repertoire, resulting in a low frequency of detectable de novo mutations. The higher frequency of mutations within NP 366 could result from the D b NP 366 + CTLs imposing more immune pressure than the D b PA 224 -specific effectors. Overall, the D b NP 366 + CD8 + population is of lower pepMHCI avidity than the D b PA 224 -specific set, with the consequence that shorter TCR contact time may lead to the lysis of greater numbers of infected targets [42] . Furthermore, vaccination with the PA 224 peptide [43] or with DCs pulsed with PA 224 peptide [44] did not lead to any reduction in viral load, indicating that the D b PA 224 + CD8 + CTLs may be essentially non-functional when it comes to immune control. Both the NP-N5H and NP-N5D mutations resulted from a single nucleotide change at the same codon position, with the difference in relative frequency for the NP-N5H versus NP-N5D mutations reflecting that NP-N5H is at a selective advantage. At least for experimental models, codon usage, viral fitness and the efficiency of evasion from existing immune responses dictate the frequency and type of amino acid changes found in CD8 + CTL epitopes. It seems from the structural studies that reduced stability of the pepMHCI complexes is a primary factor when it comes to subverting CTL recognition. Then, with regard to influenza A viruses circulating in humans, understanding the relevant antigenic variants is essential for future vaccine development. Mice and viral infection Female C57BL/6J (B6, H-2 b ), BALB/c (H-2 d ), μMT (H-2 b ) and RAG −/− (H-2 b ) mice were bred and housed under specific pathogen-free conditions at the Department of Microbiology and Immunology, University of Melbourne. To generate primary influenza-specific CD8 + T-cell responses, 6–8-week-old mice were lightly anesthetized by inhalation of methoxyflurane and infected intranasally (i.n.) with 1 × 10 4 plaque-forming units (p.f.u.) of HKx31 (H3N2, HK) influenza A virus in 30 μl of PBS. For recall responses, mice were first primed intraperitoneally (i.p.) with 1.5 × 10 7 p.f.u. of the serologically distinct PR8 (H1N1) influenza A virus in 500 μl of PBS and challenged 6 weeks later with the HK virus. All experiments were approved and conducted under guidelines set by the University of Melbourne Animal Ethics Experimentation Committee. Identification of de novo mutations from infected lung To determine the quasi species of influenza viruses generated during influenza infection, the lungs were sampled and the virus was sequenced at day 5, 10 or 15 after infection. Lungs were perfused with 5 ml of PBS through the right atrium of the heart using a 26-gauge syringe and then processed to give single cell suspensions. The pelleted cells were resuspended in 1 ml Trizol (Invitrogen, Carlsbad, CA, USA) and RNA was extracted. RNA was then resuspended in sodium citrate buffer (Ambion, Austin, TX, USA) and stored at −80 °C. vRNA was reverse transcribed to cDNA using Sensiscript kit (Qiagen, Hilden, Germany) using Uni12 primer (5′-AGCAAAAGCAGG-3′). cDNA was then purified with MiniElute kit (Qiagen) and amplified by PCR, with each reaction containing 5 μl of cDNA and 1.5 U Taq DNA polymerase, 1 × PCR buffer, 1.5 mM MgCl 2 , 0.25 mM dNTPs, 20 pmol forward and reverse primer (NP 1014 F: 5′-ACACAAGAGTCAACTGGTGTGGATGG-3′, NP 1389 R: 5′-CCATCATCCTTATGATTTCGGTCCTC-3′, PA 493 F: 5′-GGCCACAAAGGCAGACTACACTCT-3′, PA 864 R: 5′-CATCCATCAGCAGGAATTTGGACCGC-3′) (Invitrogen) (PCR conditions: 95 o C, 5 min; 95 °C, 30 s; 57 °C, 45 s; 72 °C, 1 min, × 35 cycles, final extension of 7 min at 72 °C). Positive PCR products were ligated into pGEMT vector using T4 DNA ligase (Promega) and transformed DH5α cells were plated on Luria with Ampicillin (100 mg ml −1 ) and X-gal (Bioline) in DMSO and cultured overnight at 37 °C. Incorporation of the PCR insert was screened by classic blue-white selection. White colonies were screened by colony PCR and 5 μl of positive product cleaned with 1 ml of ExoSAP-IT (USB Corporation, Cleveland, OH, USA), using for 15 min at 37 °C and then 15 min at 80 °C. Clean products (6 μl) were then sequenced with the forward primer. Sequencing products were cleaned with DyeEx columns (QIAGEN). Products were submitted to Applied Genetic Diagnostics (AGD, Department of Pathology, University of Melbourne) and resolved by ABI3130xl capillary genetic analysers. Sequences were analysed using FinchTV (Geospiza, Perkin Elmer, Seattle, WA, USA) and translated using ExPASy translate tool (accessed from www.expasy.org ). Generation of recombinant influenza viruses Recombinant influenza viruses with selected amino-acid substitutions corresponding to natural variations within the NP 366–374 peptide (NP-N3D, NP-N5H and NP-M9L) were generated using the eight-plasmid reverse genetics system [29] , [45] . Briefly, substitutions were first incorporated by site-directed mutagenesis using PCR primers encoding selected mutations, which overlap the immunogenic peptide region, and the second primer encoding the end regions of NP/PA protein and incorporated into the pHW2000 plasmid. Recombinant mutant PCR products were digested with Bsm B1 (New England Biolabs, Ipswich, MA, USA) and ligated into the alkaline phosphatase treated pHW2000 vector. Recombinant HK and PR8 viruses were rescued following transfection of MDCK-293T cell co-culture with the eight plasmids encoding influenza segments [29] . Viruses were then amplified in the allantoic cavity of 10-day-old embryonated chicken eggs and the viral titre of allantoic fluid determined by plaque assay infecting monolayers of MDCK cells. To confirm the introduction of the specific mutations within NP 366 and PA 224 , the sequences of the corresponding full-length influenza genes were assessed by extracting vRNA from allantoic fluid, followed by RT–PCR of the region of interest and sequenced. Tissue sampling and cell preparation To evaluate influenza-specific CD8 + T-cell responses following influenza virus infection, inflammatory cells were recovered from the site of infection by BAL and from secondary lymphoid organs, represented by the spleen. BAL samples were incubated on plastic petri-dishes for 1hr at 37 °C to remove macrophages. Spleens were disrupted and enriched for CD8 + T cells using goat anti-mouse IgG and IgM antibodies (Jackson ImmunoResearch Labs, West Grove, PA, USA). Cells were washed and resuspended either in cRPMI for an ICS assay or FACS buffer (1% BSA/0.2%NaN 3 in PBS) for flow cytometric analysis. Peptide stimulation and intracellular cytokine staining Lymphocytes were stimulated with wt or mutated NP 366 (ASNENMTEM) or PA 224 (SSLENFRAYV) peptides for 5 h at 37 °C, 5% CO 2 in the presence of 1μg ml −1 Golgi-Plug (BD Biosciences) and 10 U ml −1 recombinant human IL-2 (Roche Diagnostics, Basel, Switzerland). Cells were washed twice with FACS buffer, stained with anti-CD8-PerCPCy5.5 for 30 min on ice, then fixed and permeabilised using the BD Cytofix/Cytoperm Plus Fixation/Permeabilisation Kit (BD Biosciences). Cells were stained with anti-IFN-γ-FITC, anti-TNF-α-APC and anti-IL-2-PE mAbs. In selected experiments, splenocytes were stimulated with varying concentrations of peptides, threefold dilutions ranging from 300 nM to 0.0008, nM to determine sensitivity (that is, ‘functional avidity [46] ) for specific peptides. Samples were acquired using flow cytometry on a FACS Calibur and analysed with FlowJo software. The total cytokine production was calculated by subtracting background fluorescence using ‘no peptide’ controls. Hybridoma LacZ assay LacZ-inducible T cell hybridomas specific for the NP 366 peptide were incubated in 96-well flat-bottom plates together with naive splenocytes [18] , [30] . Cells were cultured in the presence of wt or mutant NP 366 peptide at concentrations ranging from 10 −14 M to 10 −4 M for 18 h at 37 °C. Cells were then washed with PBS, fixed with 100 μl of 2% formaldehyde/0.2% glutaraldehyde in PBS for 5 min on ice, washed in PBS and incubated with 2.5 mg of 5-bromo-4-chloro-3-indolyl β-D-galactoside (X-gal) for 16 h at 37 °C. The LacZ + hybridomas were then counted and the number of NP 366 -responding cells was calculated by subtracting the background LacZ expression for cells cultured in the absence of the peptide. Measuring lung viral titres Naive mice were infected i.n. with 1 × 10 4 p.f.u. of the wt HK virus. Lungs were sampled on d5, 10 or 15 after infection, homogenized, suspension was clarified by centrifugation and the virus-containing supernatant was harvested. Titres of infectious virus in the lung supernatants were determined by standard plaque assay on monolayers of MDCK cells. RNA sequencing of human viral isolates Longitudinal influenza viral isolates obtained from an immunocompromised patient [13] were stored and subsequently sequenced at the WHO Collaborating Centre for Influenza Research in Melbourne. RNA was extracted from nasopharyngeal aspirate and MDCK1 isolates using Qiamp Viral RNA mini kit (Qiagen). Reverse transcription was carried out using Thermoscript RT–PCR System for first-strand cDNA Synthesis (Invitrogen) according to the manufacturer’s recommendation with a universal primer, and the resulting cDNA (5 μl each) was subjected to PCR amplification of the NP and MP genes using Platinum Taq DNA polymerase high-fidelity and gene-specific primers (NP primers: A-NP-F1-M13F: 5′-TGTAAAACGACGGCCAGTCAGGGTWRATAATCACTCAMTG-3′; A-NP-F2-M13R: 5′-CAGGAAACAGCTATGACCAGTAGAAACAAGGGTATTTTTC-3′; M1 primers: A-MP-M13F: 5′-TGTAAAACGACGGCCAGTAGCAAAAGCAGGTAG-3′; A-MP-M13R: 5′-CAGGAAACAGCTATGACCAGTAGAAACAAGGTAGT)-3′. Sequencing of the PCR products was carried out using conventional Sanger Sequencing. Sequence assembly was performed using the SeqMan Pro module of Lasergene version 9.1.0 software (DNASTAR, Madison, WI, USA). Alignments were performed using Geneious 5.63 software (Biomatters Ltd, Auckland, New Zealand). Crystal structures and thermostability Briefly, the D b and β2-microglobulin molecules were expressed in Escherichia coli as inclusion bodies, refolded with the NP 366 peptide and its variants, then purified and crystallized [18] . The crystals were flash-frozen to a temperature of 100 K before data collection at the Australian synchrotron on the MX2 beamline with an ADSC-Q315 CCD detector. The data were processed and scaled with the XDS [47] and scaled using Scala from the CCP4 suite of programs [48] . The crystal structures were solved using the molecular replacement method with the PHASER programme [49] from the CCP4 suite of programs [48] . The search model was the structure of mouse MHC class I D b minus the peptide (Protein Data Bank accession number 3CPL) [30] . The refinement protocol used includes several cycles of refinement with PHENIX [50] and Buster followed by manual model rebuilding with Coot programme [51] . The electron densities around the peptides were unambiguous. Final refinement statistics are summarized in Supplementary Table S5 . To assess the effect of each mutation on the stability of pepMHC complexes, thermal shift assays were performed for D b NP-N5D, D b NP-N3D and D b NP-N5H. The fluorescent dye Sypro orange was used to monitor protein unfolding [52] . The thermal stability assay was performed in the Real Time Detection system (Corbett RotorGene 3000), originally designed for PCR. Each pepMHC complex was in 10 mM Tris-HCl (pH 8), 150 mM NaCl, tested at two concentrations (5 and 10 mM) in duplicate and heated from 29 °C to 90 °C with a heating rate of 1 °C min −1 . The fluorescence intensity was measured with excitation at 530 nm and emission at 555 nm. The Tm, or thermal melt point, represents the temperature for which 50% of the protein is unfolded, with the result being summarized in Supplementary Table S5 . Accession codes: The final coordinates of novel structures have been deposited with the Protein Data Bank under accession numbers: 4L8D for D b NP-N5D, 4L8C for D b -NPN3D and 4L8B for D b NP-N5H. RNA sequencing data have been deposited in the European Nucleotide Archive under accession codes: HG455022 for Matrix1 (M1) wild-type clone 19997; HG455023 for M1 wild-type clone 91097; HG455024 for M1 wild-type clone 261197-3; HG455025 for M1 mutant I131L; HG455026 for M1 I131L; N133S; T146A mutant; HG455027 for Nucleoprotein (NP) wild-type; HG455028 for NP-S2P; HG455029 for NP-N3D; HG455030 for NP-M9L; HG455031 for NP-N5H; HG455032 for NP-N5H/E7A; HG455033 for NP-N5H/E7G; HG455034 for NP-E4D/N5L; HG455035 for NP-A1T/N5H; HG455036 for NP-N5D; HG455037 for Polymerase acidic (PA)-R7K HG455038 for PA-R7T. How to cite this article: Valkenburg, S. A. et al. Acute emergence and reversion of influenza A virus quasispecies within CD8 + T cell antigenic peptides. Nat. Commun. 4:2663 doi: 10.1038/ncomms3663 (2013).